Mechanism of supercooled droplet freezing on surfaces Understanding ice formation from supercooled water on surfaces is a problem of fundamental importance and general utility. Superhydrophobic surfaces promise to have remarkable 'icephobicity' and low ice adhesion. Here we show that their icephobicity can be rendered ineffective by simple changes in environmental conditions. Through experiments, nucleation theory and heat transfer physics, we establish that humidity and/or the flow of a surrounding gas can fundamentally switch the ice crystallization mechanism, drastically affecting surface icephobicity. Evaporative cooling of the supercooled liquid can engender ice crystallization by homogeneous nucleation at the droplet-free surface as opposed to the expected heterogeneous nucleation at the substrate. The related interplay between droplet roll-off and rapid crystallization is also studied. Overall, we bring a novel perspective to icing and icephobicity, unveiling the strong influence of environmental conditions in addition to the accepted effects of the surface conditions and hydrophobicity. Understanding the icing mechanisms on surfaces [1] , [2] , [3] exposed to different environmental conditions is crucial to a broad range of applications such as power transmission lines and aerodynamic surfaces from aviation to wind turbine industries [4] , [5] . Ice accumulation on aerodynamic wing structures, for example, can cause hazardous air flow conditions, increasing drag and degrading the controllability of an aeroplane. Typically, supercooled water on a solid surface is expected to freeze with heterogeneous nucleation of ice near the water–solid interface because the roughness asperities on the substrate reduce the activation energy of heterogeneous nucleation compared with homogeneous nucleation in water [6] . Substrate heating and coatings with anti-icing chemicals have been used with partial success in tackling the commonly occurring frosting problem. Recently, use of superhydrophobic surfaces has also been proposed [7] , [8] , [9] , [10] , [11] . Because of outstanding water repellency, these surfaces have an extra advantage of being able to minimize ice accretion and adhesion. The role of surface roughness of superhydrophobic surfaces on the icephobic behaviour of the same has also been critically questioned [11] , [12] . For example [12] , it was established recently that hydrophilic surfaces with nanometer (nm)-scale roughness (smaller than the size of the first stable ice nuclei) and higher wettability display, up to an order of magnitude, longer freezing delays compared with typical superhydrophobic surfaces with larger hierarchical roughness and very low wettability. In practice, the efficacy of anti-icing materials can also be limited by the presence of frost on the surface [13] , [14] . We show that environmental humidity and gas flow, which are naturally present in a plethora of icing applications, can fundamentally alter the ice crystallization mechanism on supercooled superhydrophobic surfaces, thereby also drastically affect their icephobic behaviour and relevance. It is demonstrated that the local evaporative cooling of the liquid can render homogeneous nucleation at the free surface the thermodynamically preferred ice formation mechanism, instead of the expected heterogeneous nucleation due to contact with the substrate. We bring a new perspective to ice formation on surfaces by emphasizing the strong influence of environmental conditions over the commonly accepted effect of the surface conditions and hydrophobicity. The change in nucleation mode is explained using nucleation theory combined with the analysis of the temperature variation and evaporation of the supercooled droplet. The investigated substrates include two different hydrophobic and two different superhydrophobic surfaces. The shearing external gas flow can also induce runback of supercooled droplets along surfaces, which can have a dramatic impact on the ice formation, freezing characteristics, and thus on the overall efficiency and effectiveness of employed materials. The roll-off and break-up of the supercooled droplets on substrates were therefore investigated under nitrogen flow with controlled humidity and in the presence of substrate contamination by ice crystals. The observed humidity-dependent break-up, stickiness and roll-off of droplets on substrates were investigated using high-speed visualization, velocimetry and inertia-capillary force analysis of the supercooled droplets. Surface properties The present work aims at advancing our fundamental understanding of ice formation from supercooled water on surfaces. Freezing of supercooled sessile water droplets in a chamber with controlled gas flow and humidity provides a convenient and repeatable setting for such an investigation. The tests were performed in a dual layer flow chamber with optical access, as described in the Methods section. Four different surfaces, with wettability ranging from hydrophobic to superhydrophobic, were tested in the presence of a shearing nitrogen flow at a chamber temperature of −15 °C. Four different chamber humidities of unsaturated (relative humidity φ : 30, 60 and 75%) and saturated ( φ =100%) states were used to examine the influence of humidity. The experiments were initiated after reaching thermal equilibrium (−15 °C) by turning on the nitrogen gas flow. 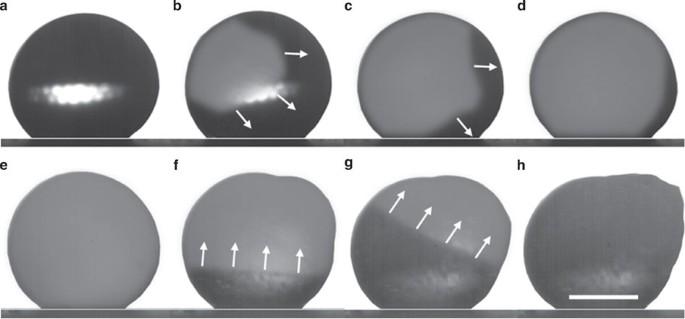Figure 1: Freezing of a supercooled water volume under shear flow. First (a–d, showing snapshots at 6 ms interval) and second phases (e–h, showing snapshots at 0, 5, 9, 13 s) of crystallization of a 5-μl droplet on a superhydrophobic surface in an unsaturated nitrogen flow field (flow direction from left to right). The origin and direction of the arrows, respectively, mark the instantaneous position and direction of motion of the freezing front. The scale bar equals 1 mm. Table 1 lists the roughness parameter ( R a value), measured using confocal laser scanning microscopy, described in the Methods section, wettability parameters and critical gas velocities causing droplet roll-off/sliding for the tested surfaces. Table 1 Characteristics of the four tested surfaces. Full size table For a sessile droplet exposed to gas flow, the downstream contact angle (advancing side) was higher than the upstream receding side. The difference between the advancing and the receding contact angles is referred to as contact angle hysteresis (CAH) [15] , [16] . The critical shear flow velocity, U crit , for the onset of droplet roll-off/sliding depends on factors such as the drop shape, properties and substrate wettability. The later can be quantified in terms of the static water contact angle by assuming a spherical cap-like geometry for the droplet on the substrate. Droplets on superhydrophobic surfaces (that is, surfaces 1 and 2 in Table 1 ) have high contact angle, low CAH and relatively large frontal area exposed to shearing gas flow resulting in stronger drag force. Therefore, U crit for droplet roll-off/sliding on superhydrophobic surfaces was lower than for smooth, hydrophobic surfaces with lower contact angle, higher CAH and smaller frontal area (for example, surface 3 and 4 in Table 1 ) [15] . For suitably designed superhydrophobic surfaces, air pockets can be trapped below the water drop (Cassie state), which results in reduced CAH and less sticking [16] . The opposite effect is observed in the Wenzel state, where the water penetrates and gets locked in surface asperities, thereby resulting in high CAH and droplet adhesion, even though the contact angle is high [16] . The Wenzel state is especially common on surfaces with lower roughness (for example, surface 3). It can also become dominant for a superhydrophobic surface exposed to a supersaturated environment, where condensed water can replace the air in the rough surface texture [16] . A droplet placed on such a surface is in contact with water trapped on the surface, which leads to a significant increase in the CAH [16] and U crit (see Table 1 measurements for surfaces 1 and 2 at φ =100%). The CAH for surface 3 (the smoother, slightly hydrophobic surface) remained almost unaffected by humidity due to the lack of trapped air pockets. Nucleation mechanisms After the characterization of the substrates, ice nucleation of a supercooled sessile water droplet placed on them was investigated by subjecting the droplets to nitrogen shear flow under different humidity conditions. Figure 1 shows a typical image sequence capturing the location of nucleation (near the gas–liquid interface) and the subsequent crystallization process on a superhydrophobic surface (surface 2) in an unsaturated environment ( φ =30%). Similar nucleation and freezing mechanisms were also observed for surface 1. The freezing process for a supercooled droplet, with or without the presence of shearing gas flow, proceeded in two sequential stages [17] and was initiated by either spontaneous homogeneous nucleation near the gas–liquid interface or spontaneous heterogeneous nucleation at the liquid–substrate interface. The supercooled droplet in Figure 1 was subjected to shearing gas with a free-stream velocity of 3 m s −1 , that is, slightly under U crit as per Table 1 . The image sequence for the no-flow case is shown in Supplementary Figure S1 and discussed in Supplementary Note 1 . During the first stage, a very rapid, recalescent, partial solidification of the droplet takes place during which most of the released latent heat of fusion is absorbed by the liquid raising its temperature, while only a small portion is transferred to the surroundings. This rapid kinetically controlled process can be recognized in Figure 1a–d through a gradual clouding of the water volume, starting from the point of nucleation. In the second stage ( Fig. 1e–h ), the remaining liquid freezes isothermally at a rate nearly three orders of magnitude slower than the first stage. The freezing in this stage is controlled by the rate of heat conduction to the substrate and dissipation to the environment by convection resulting in a freezing front, which always starts from the droplet–solid interface and grows upwards. The important and interesting finding here is that the freezing process presented in Figure 1 starts with homogeneous nucleation at the gas–liquid interface ( Fig. 1a–d ), instead of the commonly expected heterogeneous nucleation [18] at the liquid–solid interface for supercooled droplets in the absence of shear flow from unsaturated ( φ =30%) gas. The nucleation mode is clearly visible in Supplementary Movies 1 and 2 (ref. 12 ). In Figure 1 , the origin and direction of the arrows mark the instantaneous location and direction of the freezing front. The homogeneous nucleation observed for 'dry' humidity conditions was highly reproducible. The result is of central importance in deciding the efficacy of anti-icing coatings, because an otherwise well-performing coating can be rendered entirely ineffective, if the freezing starts away from liquid–solid interface owing to a gas velocity or humidity change. Additional experiments, presented in Supplementary Figure S2 and Supplementary Note 2 , at even higher humidity values of 60 and 75%, further confirmed the occurrence of homogeneous nucleation on the superhydrophobic samples 1 and 2. The reason for the homogeneous nucleation process, described above, can be understood by considering the heat transfer physics of the droplet. Figure 1: Freezing of a supercooled water volume under shear flow. First ( a–d , showing snapshots at 6 ms interval) and second phases ( e–h , showing snapshots at 0, 5, 9, 13 s) of crystallization of a 5-μl droplet on a superhydrophobic surface in an unsaturated nitrogen flow field (flow direction from left to right). The origin and direction of the arrows, respectively, mark the instantaneous position and direction of motion of the freezing front. The scale bar equals 1 mm. Full size image A supercooled water droplet in an unsaturated gas will undergo evaporation, which reduces the liquid temperature locally, at the gas–liquid interface. We determined the evaporation rate of the droplets on surfaces in the absence of any gas flow. The detailed derivation can be seen in Supplementary Methods . The temperature reduction under flow conditions is of course higher than that for no-flow, pure diffusive evaporation, under which nucleation always takes place at the liquid–solid interface [12] . The evaporation rate will be higher at the upstream region of the interface, when the droplet is subjected to shear flow. This will lead to a higher temperature reduction and more probable ice nucleation at the upstream region of the gas–liquid interface. In the following, the temperature differential at the gas–liquid interface is estimated for a sessile droplet placed on a superhydrophobic surface for pure diffusion and convection conditions. For the latter, an average gas velocity value, U g , of 2 m s −1 is used to account for the velocity variation in the boundary layer. Under quasi steady-state conditions, the energy balance at the gas–liquid interface of an evaporating droplet can be obtained by equating the energy required for evaporation, Q̇ v , to the sum of the energy transferred by convection from the surrounding gas, Q̇ g , and heat conduction from the droplet bulk to the interface, Q̇ w , as In writing equation (1), we have neglected the heat transfer at the solid–liquid interface. This is justified because we allow enough time, as described in Methods section, for the droplet to cool down to the chamber and substrate temperatures before placing it on the substrate. By making appropriate substitution for the different terms in the equation above, including a realistic correlation to determine the convective heat transfer coefficient at the gas–liquid interface of the droplet, we can estimate the local temperature differential at the gas–liquid interface of the water droplet as where Δ H , ρ , M , h , k , l , r denote the enthalpy of vapourization, the density, the molecular weight, the convective heat transfer coefficient, the thermal conductivity, the height and the radius of the droplet, respectively. The subscripts v, g, w denote water vapour, gas and liquid water, respectively, and the subscript 0 is used to denote the initial value of a parameter. The evaporation rate constant ξ was experimentally determined, as described in Supplementary Methods and Supplementary Figure S3 , separately for flow and no-flow conditions. The derivation of equation (2) is provided in the Supplementary Methods . A temperature differential Δ T =0.34 K was obtained for the forced convection case and a negligibly small Δ T =0.02 K was obtained for the case of no external flow. Comparison of both values of Δ T shows the clear influence of convection of heat under shearing gas flow. It can be argued that, if this local reduction in the temperature is large enough, homogeneous nucleation near the gas–liquid interface could become thermodynamically more favourable compared with the heterogeneous nucleation at the liquid–solid interface. To pursue this critical argument, we need to compute the free energy barriers for homogeneous and heterogeneous nucleation to determine the required temperature reduction. Following Fletcher [19] , the free energy barrier for heterogeneous nucleation around a spherical particle of radius R is reduced by a factor f (ranging from 0 to 1) compared with that for homogeneous nucleation: with where γIW is the water–ice interfacial tension [20] and is the volumetric free energy difference between the bulk ice and the bulk liquid, which follows from the Gibbs–Helmholtz equation; Δ Hf,v is the volumetric enthalpy of fusion [20] ; and Tw and T m are the water droplet temperature and the melting point of ice at one atmosphere ( ∼ 0 °C), respectively. Tw can be determined from the Δ T estimated earlier. The water droplet static contact angle, θ , the nominal size of surface roughness, R s , and the critical ice nucleus radius (that is, the minimum size an incipient ice crystal needs to reach to maintain a stable freezing process), rc [19] , are the principal parameters determining the factor f in equation (3). The roughness parameter can be better appreciated by seeing the scanning electron microscope image in Supplementary Figure S4 . For a ratio the heterogeneous nucleation process depends primarily on θ (ref. 19 ) and the wetting parameter f can be expressed as [12] , [21] where γ I , γ W denote the ice–gas, and water–gas interfacial tensions, respectively [20] . 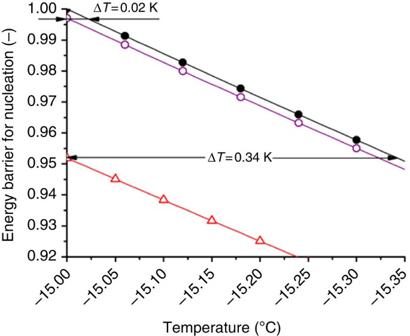Figure 2: Nucleation energy barrier versus temperature. Energy barriers for homogeneous and heterogeneous nucleation for different water temperatures and two different substrate wettabilities (contact angles). Black line with filled circle markers: homogeneous nucleation; purple line with open circle markers: heterogeneous nucleation (for surface 2,θ=145°); red line with open triangle markers: heterogeneous nucleation on a hypothetical surface withθ=130° for which the nucleation should switch back to the heterogeneous mode even with evaporative cooling. The energy barrier values are normalized with the energy barrier for homogeneous nucleation at −15 °C. Using the contact angle for surface 2 in Table 1 , the free energy barriers for homogeneous (calculated using equation (4)) and heterogeneous nucleation (calculated using equation (3)) are plotted as a function of the water temperature Tw in Figure 2 . The energy values were normalized with the energy barrier for homogeneous nucleation at −15 °C for comparing the relative magnitudes. It is clear from Figure 2 that, with no gas flow, the droplet temperatures near the solid–liquid and gas–liquid interfaces differ only by 0.02 K, and the critical energy barrier for heterogeneous nucleation remains lower than that for homogeneous nucleation. Therefore, for a supercooled droplet on a substrate without any external shear gas flow, heterogeneous nucleation at the solid–liquid interface should typically initiate freezing. This was confirmed in all our experiments on superhydrophobic surfaces without external gas flow. Figure 2: Nucleation energy barrier versus temperature. Energy barriers for homogeneous and heterogeneous nucleation for different water temperatures and two different substrate wettabilities (contact angles). Black line with filled circle markers: homogeneous nucleation; purple line with open circle markers: heterogeneous nucleation (for surface 2, θ =145°); red line with open triangle markers: heterogeneous nucleation on a hypothetical surface with θ =130° for which the nucleation should switch back to the heterogeneous mode even with evaporative cooling. The energy barrier values are normalized with the energy barrier for homogeneous nucleation at −15 °C. Full size image Recalling the temperature difference of Δ T =0.34 K under flow conditions, the water temperature at the gas–liquid interface is reduced down to −15.34 °C. Therefore, the energy barrier for homogeneous nucleation is well below the heterogeneous nucleation, which explains the observed homogeneous nucleation under flow conditions. The energy barrier for heterogeneous nucleation on a hypothetical surface with θ= 130 ° is also plotted with open triangles in Figure 2 to illustrate the influence of wettability change on energy barriers. Because of the water contact angle reduction from 145 to 130°, the energy barrier for heterogeneous nucleation again becomes lower than that for homogeneous nucleation even under forced convection. The switchback to heterogeneous nucleation owing to a contact angle reduction (for example, on surfaces 3 and 4), as well as further experiments confirming the effect of environmental humidity, is discussed in more detail in the Supplementary Note 2 and 3 , and Supplementary Figures S2 , S5 and S6 . The above discussion establishes the influence of evaporative cooling on the ice nucleation mechanism. As the evaporation process is humidity dependent, the influence of humidity on the nucleation process must be investigated. To this end, at constant gas velocity and temperature, and under the assumption of a quasi-steady evaporation, the evaporation rate coefficient ξ can be expressed as the sum of contributions due to diffusion [22] and convection where φ denotes the relative humidity expressed as fraction and the symbols D and ρv,sat , respectively, denote the diffusivity of water vapour in air and the saturated water vapour mass concentration at the gas–liquid interface. The parameter C accounts for the influence of gas flow on the droplet. We determined ξ for φ =30%, through separate experiments, recording the change in droplet volume due to evaporation with and without gas flow. The droplet volume change with time was obtained by processing the digitized image sequence of the video recording of the droplet evaporation, which is described further in the Supplementary Methods . The values of ξ determined were used to obtain the constant C in equation (6). From equations (2) and (6), the interface temperature difference due to evaporation, as a function of the relative humidity, can be obtained. Clearly, this temperature difference can be significantly reduced by increasing the humidity of the flowing gas, thereby resulting in a reversal of the nucleation process from homogeneous to heterogeneous nucleation. For example, at humidity φ =95%, the corresponding temperature difference comes out to be negligibly small, Δ T =0.02 K. This was confirmed by running experiments in several differently controlled humidity conditions (more details are given in the Supplementary Note 2 ), where, indeed, we observed heterogeneous nucleation even in the presence of shearing flow at saturated conditions. It is worth stating that the above, although approximate, does contain all essential elements of the physics of the problem and underpins the important finding that the humidity-dependent evaporation rate influences the generated temperature differential at the droplet surface, which in turn, affects the nature of ice nucleation, switching from the homogeneous to the heterogeneous mode and vice versa. Droplet roll-off, stickyness and pinch-off A superhydrophobic surface is expected to facilitate easy roll-off of supercooled water droplets in the presence of flow, thereby minimizing the problem of ice accumulation in practical applications. However, the roll-off behaviour is likely to be strongly influenced by ambient humidity. We observed that the supercooled droplets on superhydrophobic surfaces (surfaces 1–2) started to move and roll-off well before freezing when exposed to sufficiently strong nitrogen flow. The roll-off starts once the adhesion force of the droplet to the surface is overcome by the drag force from the gas flow, that is, at velocity U crit , enumerated in Table 1 . For surfaces 1–2, the roll-off velocities (plotted in the Supplementary Figure S7 for two different humidity conditions) of the droplets were found to increase strongly from 'dry'-to-'wet' surface conditions (more details are given in Supplementary Note 4 ). Owing to the increased adhesion force due to water-filled asperities on these surfaces, the critical free-stream velocity and thus the relative velocity (difference between free-stream velocity and roll-off velocity of the droplet) was much higher for the 'wet' surfaces. Supplementary Figure S7 shows the variation in supercooled droplet roll-off/sliding velocity on surface 2 at the critical gas-shearing velocity for different positions of the droplet with respect to the leading edge of substrate and under two different humidity conditions. Similar results for surface 1 are not presented for brevity. In a natural environment, the solid surface is also likely to be contaminated with ice crystals that could act as nuclei initiating droplet freezing. In the following, we describe the results of our experiments to study this phenomenon on two superhydrophobic surfaces (surfaces 1 and 2). We seeded the surface with a small ice cluster in the trajectory of a rolling droplet (5 μl, droplet velocity=0.53 m s −1 , gas free-stream velocity ∼ 9 m s −1 ). 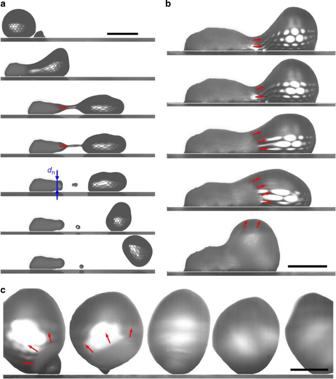Figure 3: Supercooled sessile droplets under shear. Humidity dependent pinch-off (a), stickyness (b) and roll-off (c) of supercooled droplets on superhydrophobic surfaces after encountering an ice cluster. The surface is dry in (a) and (c) and wet in (b). For sequence (a), the snapshots are times 0, 8, 12.5, 13, 13.5, 16 and 19 ms. For sequence (b), snapshots are at time 0, 2, 4, 6 and 16 ms. For sequence (c), snapshots are at time 0, 3, 7, 13 and 18 ms. The ice cluster is stuck to and loosely resting on the surface for (a,b) and (c), respectively. The blue arrows in photograph3aat Δt5indicate the crystallization front diameterdn. The flow/roll-off direction is from left to right. The origin and direction of the red arrows mark the instantaneous position and direction of the freezing front, respectively. Scale bar for sequence (a) is 2 mm, and those for sequences (b) and (c) are 1 mm. High-speed images of a shear flow-driven supercooled droplet running over an ice cluster ( ∼ 0.5 mm diameter) on a dry ( φ =30%, Figure 3a,c ) and a wet surface ( φ =100%, Fig. 3b ), showed an interesting interplay of the droplet roll-off and freezing timescales and the resulting droplet deformation. Figure 3a and Supplementary Movie 3 clearly show that, while part of the droplet rests on the frozen ice cluster and rapidly partially crystallizes (first crystallization phase described earlier), the rest of it is pinched–off by the formation of a shear flow-induced neck. It is visible in Figure 3a (Δ t 3 –Δ t 5 ) that the break-up takes place before the freezing front reaches the break-up point and thus the detached part of the droplet breaks off and departs in the liquid state (Δ t 5 –Δ t 7 ). From frame Δ t 4 to the next in Figure 3a, the neck pinches off and contracts into a satellite droplet, which is a universal behaviour of break-up of low viscosity liquids [23] . Figure 3: Supercooled sessile droplets under shear. Humidity dependent pinch-off ( a ), stickyness ( b ) and roll-off ( c ) of supercooled droplets on superhydrophobic surfaces after encountering an ice cluster. The surface is dry in ( a ) and ( c ) and wet in ( b ). For sequence ( a ), the snapshots are times 0, 8, 12.5, 13, 13.5, 16 and 19 ms. For sequence ( b ), snapshots are at time 0, 2, 4, 6 and 16 ms. For sequence ( c ), snapshots are at time 0, 3, 7, 13 and 18 ms. The ice cluster is stuck to and loosely resting on the surface for ( a , b ) and ( c ), respectively. The blue arrows in photograph 3a at Δ t 5 indicate the crystallization front diameter d n . The flow/roll-off direction is from left to right. The origin and direction of the red arrows mark the instantaneous position and direction of the freezing front, respectively. Scale bar for sequence ( a ) is 2 mm, and those for sequences ( b ) and ( c ) are 1 mm. Full size image Crucial differences existing in the timescales, involved in the two stages of freezing presented in Figure 1 for different humidity and gas flow conditions, require discussion. The differences can be interpreted in the light of the earlier analysis of the temperature differential and the influence of the flowing gas humidity as follows. First, the recalescent stage of freezing ( Fig. 1a–d ) is very rapid and is accelerated by the efficient removal of the generated heat by the unsaturated gas flow. The actual observed crystallization time was ∼ 18 ms for a droplet in forced convection (homogeneous nucleation) compared with ∼ 32 ms in the absence of external flow (heterogeneous nucleation). Second, while the crystallization front of the second—markedly slower—stage of freezing gradually moves upward starting from and parallel to the solid–liquid interface in the absence of external flow [12] . Under flow conditions, however, this front moves faster at the upstream side of the droplet than at the downstream side, because of convective cooling asymmetry. The external flow leads to an inclination of the freezing front, with respect to the solid–liquid interface, which is visible in Figure 1g , and a markedly shorter freezing time of ∼ 13 s compared with ∼ 20 s in the absence of external flow. The physics of the droplet deformation and necking phenomenon shown in the sequence of Figure 3a can be understood by estimating the relative effect of the various forces acting on the droplet represented by the capillary number, (ratio of the viscous to surface tension forces) and the Weber number, (ratio of the inertia and surface tension forces [24] ). Using the crystallization front diameter in Figure 3a (Δ t 5 ) as the characteristic length ( d n =0.5 mm), we estimated from the measurements the relative velocity of the pinching part of the droplet as where U pinch and U ice denote the velocity of the unfrozen (separating) part of the droplet and the freezing front, respectively. The relative velocity is computed using the velocities obtained by processing the image sequence of the recorded video ( U pinch ∼ 0.43 m s −1 and U ice ∼ 0.1 m s −1 ). The resulting value of We was We=0.7. These values for We and Ca point to a break-up that is similar in nature to a dripping type break-up as established by Utada et al . [24] Contrary to the break-up on a dry superhydrophobic surface in Figure 3a , no neck leading to separation is observed in Figure 3b . The droplet here sticks to the pre-wetted surface, it is simply deformed by the shear forces at the interface and freezes entirely. In a wet nanotextured surface, the water saturates air pockets owing to condensation, thereby increasing surface adhesion. The frozen part of the droplet, in contact with the ice cluster, naturally experiences strong shear-induced drag force on both dry and wet surfaces. However, the still liquid part of it moves at different rates, depending on the balance of the drag force from gas stream and the adhesive force on the solid surface due to wetting. Therefore, while on the dry surface, stronger stretching due to gas shear results in the neck formation and pinch-off due to surface tension ( Fig. 3a ), Δ t 1 –Δ t 3 ; on a wet surface, the drag included by the same external flow cannot overcome the increased substrate adhesion because of condensed water ( Fig. 3b ). The first frame of Figure 3b (Δ t 1 ) shows the maximum downstream expansion of the droplet. An interesting subset of roll-off dynamics observed on dry surfaces is presented in sequence of Figure 3c , where the ice cluster rests loosely on the surface. As the cluster is overrun by a supercooled droplet, it merges with the droplet (Δ t 1 –Δ t 2 ) and initiates the recalescent crystallization of water. The freezing droplet rolls off the surface downstream, before the second stage of crystallization could take place. In summary, supercooled (−15 °C) water droplets on surfaces with wettabilities ranging from slightly hydrophobic to superhydrophobic have been studied to evaluate the droplet freezing and motion characteristics under variable humidity and shear flow. The substrate temperature was maintained at −15 °C. On superhydrophobic surfaces, a counterintuitive and very important, humidity and gas velocity-dependent mode of crystallization was observed for unsaturated flow conditions wherein homogeneous nucleation at the gas–liquid interface and away from the solid substrate was responsible for the droplet freezing. Local evaporative cooling at the gas–liquid interface was shown to be the reason for the preferred thermodynamic state of homogeneous nucleation over the commonly observed heterogeneous nucleation due to the presence of the substrate. The conditions of a possible transition from homogeneous back to heterogeneous nucleation were also predicted by combining nucleation theory with heat transfer scaling analysis of the supercooled droplets under high environment humidity. The humidity was also shown to have a drastic effect on the roll-off/sliding of a supercooled droplet on superhydrophobic surfaces under shear flow. For a superhydrophobic surface, pre-wetted through condensation from a supersaturated ambient, the droplet adhesion increased dramatically resulting in the critical shearing gas velocity required for the onset of droplet motion to be more than twice the value for dry surfaces. Whereas, on a dry superhydrophobic surface, rolling water droplets, coming in contact with small ice crystals, either partly froze and pinched-off or entirely rolled-off, the droplet, despite shear-induced deformation, remained completely attached and froze, when the surface was wet. The present basic findings shed new light on the interplay of environmental and surface conditions on the freezing of undercooled droplets and can have serious implications on the function, performance and limitations of icephobic surfaces, a topic of great general interest and general utility. Tested surfaces Four different surfaces of varying wettability and roughness were used in our experiments. Surface 1 was a superhydrophobic coating, obtained from a commercial supplier (Fuji Heavy Industries Ltd. Aerospace Company). It is a mixture of an acrylic urethane resin and polytetrafluoroethylene (PTFE) particles coated ( Supplementary Figure S4a ) on a smooth aluminium substrate (50 mm × 50 mm × 1 mm). As per the manufacturer, the coating was primarily developed for aircraft icing prevention. More detailed information on the preparation and performance of this coating is given in Kimura et al . [25] Surface 2 is a nearly superhydrophobic surface consisting of a closely packed TiO 2 nanotube array. It was developed using an anodizing process on titanium alloy Ti 6 Al 4 V (50 mm × 50 mm × 1 mm) as substrate. The following conditioning steps were carried out prior to the pre-treatment process. The titanium alloy piece was cleaned with an alkaline cleaner P3 Almeco 18 (Henkel) at 70°C, 3°C for 15 min and then dropped in an etching bath Turco 5578 (Henkel) at 95°C, 3°C for 5 min. Then, to form the TiO 2 nanotube layer ( Supplementary Figure S4b ), the anodizing was performed using a two-electrode cell with Ti 6 Al 4 V as working electrode and Ti 6 Al 4 V as cathode. The anode to cathode ratio was 1:1 and an ammonium sulphate/ammonium fluoride mixture was used as electrolyte. The process was carried out under a constant applied voltage at 25°C. The anodized substrate was washed thoroughly with deionized water and dried using nitrogen. Subsequently, the surface was treated with fluorosilane (Dynasylan F 8261, Degussa). The silane was hydrolysed for 2 h by mixing it with water and isopropanol in the weight ratio of isopropanol/F8261/water=93/2/5. The surface was dip-coated for 2 min in the silane solution and subsequently rinsed with deionized water for 30 s and finally heated at 80°C for 1 h. Note that although the measured contact angle for surface 2 is slightly less than 150°, the low value of CAH for this surface justifies referring to it as self-cleaning superhydrophobic surface. The same is also true for surface 1. Surface 3 was an untreated polytetrafluoroethylene (PTFE) foil (50 mm × 50 mm × 1 mm, Ammerflon GmbH, Germany) applied on a smooth aluminium substrate. Surface 4 'PhaseBreakTM ESL' (50 mm × 50 mm × 1 mm) was obtained from a commercial supplier (MicroPhase Coating, Inc.). It was synthesized to have icephobic properties by including different salts (e.g. ethoxy silicates) acting as freezing point depressants. Surface characterization The static contact angle and the contact angle hysteresis ( Table 1 ) of a supercooled sessile droplet (5 μl) were measured using a drop shape analysis system (Kruess G10/DSA10). Roughness measurements were carried out using a confocal laser scanning microscope (Olympus Lext OLS 3100). The roughness R a values, listed in Table 1 , were obtained in non-contact mode and are the arithmetic average of the roughness profile obtained from five measurements, each at different locations. 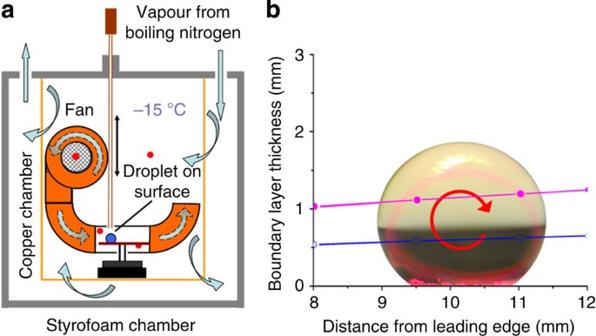Figure 4: Test set-up. (a) Schematic of the experimental set-up showing the wind tunnel inside the inner chamber. The red dots indicate the thermocouple locations. (b) Initial configuration of a sessile drop subjected to shear gas flow at room temperature. The red ellipse and the red circular arrow, respectively, indicate the visualized trajectory and direction of the moving seed particles. The calculated boundary layer dimensions for maximum (11 m s−1, pink lines with filled circle markers) and minimum (3 m s−1, blue lines with open circle markers) free stream velocities are also shown. Experimental procedure and apparatus A double-wall chamber shown schematically in Figure 4a , with the inner and outer walls made from copper and styrofoam, respectively, was used for performing the experiment. The styrofoam outer layer helped minimize the heat loss during experiments and the copper box helped control the cold nitrogen vapour flow as well as the chamber temperature. A double layer glass pane in the front of the box was used for optical access to the droplet under test. The detailed dimensions and design of the experimental chamber were described elsewhere [12] . Figure 4: Test set-up. ( a ) Schematic of the experimental set-up showing the wind tunnel inside the inner chamber. The red dots indicate the thermocouple locations. ( b ) Initial configuration of a sessile drop subjected to shear gas flow at room temperature. The red ellipse and the red circular arrow, respectively, indicate the visualized trajectory and direction of the moving seed particles. The calculated boundary layer dimensions for maximum (11 m s −1 , pink lines with filled circle markers) and minimum (3 m s −1 , blue lines with open circle markers) free stream velocities are also shown. Full size image The double-wall chamber set-up was fitted with an open low-speed wind tunnel (3–11 m s −1 ) to regulate the gas flow on the freezing droplet under test. The wind tunnel consisted of a fan (Karl Klein GmbH, ENG 1–1.5), which fed cool nitrogen gas to the U-shaped tunnel. To minimize the fluctuation in the gas velocity, the gas stream was linearized by passing through a honeycomb type flow straightener and then guided into the tunnel test section using guide plates. The test section was made of plexiglass for visual access to the droplet under test. A second set of guide plates at the downstream side of the plexiglass test section turn the nitrogen gas back into the open part of the inner chamber. The plate samples were placed on an automated rotary stage (Micro Control-ITL09) fitted inside the test section. The plate samples were positioned centrally with respect to the test-section cross-section (50 mm×60 mm). The water droplets (deionized water, ∼ 5 μl) were deposited ∼ 10 mm downstream from the leading edge on the surfaces ( Fig. 4a,b ), using a pipette after cooling the droplet down to the test-section ambient temperature (−15 °C). The temperature was lowered by letting the droplet hang from the polypropylene pipette (electronic repetitive pipette Handystep, Brand GmbH & CoKG) at ∼ 3 cm from substrate before depositing it on the surface. Supplementary Methods and Supplementary Figure S8 provide details for the estimation of this waiting time. Under normal conditions, φ was 30%. The nozzle of a piezo-electric nebulizer (with a flow rate of 500 mg min −1 and a median droplet size of <4 μm diameter) was connected to the inner chamber of the setup to control the relative humidity values in the range 30%–100%. In order to adjust the corresponding humidity, water from the reservoir of the nebulizer was gradually injected into the chamber volume (0.05 m 3 ) until the humidity of circulating nitrogen gas reached equilibrium. The humidity was measured using a humidity sensor (see below) and calibrated with the amount of water atomized into the chamber. For running tests in the saturated humidity conditions, a small amount of water was condensed on the sample surface by replacing the nitrogen of the inner chamber with supersaturated air (330±3% at −15 °C). After the ambient gas, the sample surface and the deposited water droplet temperatures reached −15±0.3 °C, the nitrogen gas flow was gradually increased using the ventilation to desired levels. To repeat any experiment on a sample, in between two successive experiments, the sample was turned by the rotary stage by 90° to ensure similar surface conditions for each droplet. The temperature was monitored using K-type thermocouples (red dots in Fig. 4a ). The first thermocouple (T1) was located immediately next to the inlet of the ventilation unit. Thermocouples T2 and T3 were placed near the test sample and in the middle of the inner chamber, respectively. The reading from T2 was used to control the temperature using a feedback control unit [12] . T4 was attached directly onto the sample surface downstream from the droplet location. The relative humidity was measured and controlled using a humidity sensor (Graphtec, B-530), located downstream of the test section. A pitot tube (PCE-Instruments, PCE-DM-2L) was used to correlate the variation of the gas stream velocity at the centre of the test section to the fan rotation speed. The calibration results are shown in the Supplementary Figure S9 . The measured velocity at −15 °C was used as free-stream velocity U ∞ and, to estimate the size of the boundary layer on the sample surface, the Blassius solution [26] was used. The result is plotted in Figure 4b for two different velocities. Water and nitrogen viscosities differ by almost three orders of magnitude. This should lead to the formation of a shear layer at the gas–water interface and thus to an internal recirculation inside the droplet. To visualize this internal motion, the sessile water droplet was seeded with PMMA particles at room temperature (microparticles GmbH, PMMA-RhB-FRAK-B1430, 20–50 μm diameter, ∼ 115 particles μl −1 ) , and the flow circulation were monitored by high-speed imaging. The experiment was performed at −15 °C. Figure 4b shows a typical example of flow recirculation observed inside the droplet at a shearing gas speed of 3 m s −1 . The velocity of a single particle was evaluated from a PIV (particle image velocity) analysis of two consecutive frames. Unlike the usual bidirectional symmetric circulation observed inside a falling water droplet in air or the Marangoni flow inside a sessile water droplet evaporating on a surface [20] , [27] , only one direction of circulation is visible in Figure 4b because of the asymmetric shear flow around the sessile droplet [28] . High-speed recordings were made through the observation window using a high-speed camera system (Photron Fastcam PCI1024) with a maximum image resolution of 1,024×1,024 pixels, mounted on a binocular microscope (Olympus SZX10). How to cite this article: Jung, S. et al . Mechanism of supercooled droplet freezing on surfaces. Nat. Commun. 3:615 doi: 10.1038/ncomms1630 (2012).